Sulphur shuttling across a chaperone during molybdenum cofactor maturation Formate dehydrogenases (FDHs) are of interest as they are natural catalysts that sequester atmospheric CO 2 , generating reduced carbon compounds with possible uses as fuel. FDHs activity in Escherichia coli strictly requires the sulphurtransferase Ec FdhD, which likely transfers sulphur from IscS to the molybdenum cofactor (Mo- bis PGD) of FDHs. Here we show that Ec FdhD binds Mo- bis PGD in vivo and has submicromolar affinity for GDP—used as a surrogate of the molybdenum cofactor’s nucleotide moieties. The crystal structure of Ec FdhD in complex with GDP shows two symmetrical binding sites located on the same face of the dimer. These binding sites are connected via a tunnel-like cavity to the opposite face of the dimer where two dynamic loops, each harbouring two functionally important cysteine residues, are present. On the basis of structure-guided mutagenesis, we propose a model for the sulphuration mechanism of Mo- bis PGD where the sulphur atom shuttles across the chaperone dimer. In the context of limited fossil fuel resources and because of the need to restrict emissions of CO 2 , the main green-house gas, it is essential to develop research for CO 2 valourization. One of the most promising ways is to transform CO 2 into more reduced forms of carbon that can then be used to generate hydrocarbons. The major difficulty lies in the fact that CO 2 is a very stable compound, which is difficult to activate chemically. However, the microbial formate dehydrogenases (FDHs) are able to perform the reversible reduction of CO 2 into formate in mild conditions with a high efficiency [1] , [2] . Only few FDHs have been characterized as formate-producing enzymes, most of those identified so far being formate consumers [3] . However, both types of enzymes share high sequence similarity and their reaction can be efficiently reversed by electrocatalysis [4] . FDHs are mononuclear molybdenum (Mo)- or tungsten (W)-containing enzymes belonging to the dimethyl sulphoxide reductase family, an ancient and widespread family in prokaryotes [5] , [6] . Crystallographic structures indicate that the active site of FDHs in the oxidized state contains either an Mo or a W ion hexacoordinated to four sulphur atoms from two pyranopterin molecules linked to a GDP nucleotide, one selenium atom from a selenocysteine (SeCys), and an additional inorganic sulphur atom [7] . The additional sulphur is also found in the Mo coordination sphere of periplasmic nitrate reductases, as well as in members of the xanthine oxidase family [8] , [9] . Most interestingly, this inorganic sulphur is crucial for the activity of both FDHs and members of the xanthine oxidase family, while its functional significance in periplasmic nitrate reductases remains to be established [10] , [11] . In Escherichia coli , the FDH activity requires the protein FdhD that was reported to act as a sulphurtransferase between the L -cysteine desulphurase IscS and FDHs [11] . Residues Cys121 and Cys124 of Ec FdhD have been shown to be involved in this reaction. The current working model predicts that Cys121 is the catalytic residue involved in both sulphur transfer from IscS to Ec FdhD and FDH activation, while Cys124 of Ec FdhD promotes sulphur release from the persulphurated Cys121 residue to the terminal sulphur acceptor, the cofactor Mo- bis PGD (Molybdo- bis (pyranopterin guanine dinucleotide)). As persulphides are generally highly reactive, Ec FdhD likely possesses a sophisticated mechanism to ensure modification of Mo- bis PGD at the correct position. However, the catalytic mechanism of molybdenum cofactor sulphuration in FDHs, as well as members of the xanthine oxidase family and periplasmic nitrate reductases is still unknown. The question has been difficult to address because the molybdenum cofactor is oxygen sensitive, very labile and never found in its free state. Moreover, three-dimensional (3D) structures of molybdoenzymes demonstrate that it is systematically found buried in the enzyme. For instance, in E. coli FdhF, the cofactor is 25 Å away from the enzyme surface, thus rendering it inaccessible to Ec FdhD [12] . This suggests that the cofactor is likely sulphurated prior to its insertion in the apoenzyme. Interestingly, the structure of an FdhD homologue in the δ-proteobacteria Desulfotalea psychrophila has been solved ( Dp FdhD; pdb code 2PW9, unpublished) and revealed that it has structural homologies with the cytidine deaminase family of nucleotide-interacting proteins [13] . As nucleotides are chemical moieties of the Mo- bis PGD structure [14] , it has been hypothesized that Ec FdhD could bind and sulphurate the cofactor before its insertion into FDHs [11] . A recent study supports this hypothesis with the copurification of Mo- bis PGD onto FdsC, an FdhD homologue from Rhodobacter capsulatus [15] . In this study, we present structural and functional data that provide a basis for molybdenum cofactor sulphuration catalysed by the FdhD family. We confirm that Ec FdhD copurifies with Mo- bis PGD in vivo and shows that it interacts at a submicromolar affinity with GDP in vitro . The Ec FdhD crystal structure was solved in complex with GDP showing a dimer that contains an empty tunnel-like structure at its centre that connects two opposite faces of the dimer. Two conserved cysteine residues (Cys121 and Cys124) are part of a disordered loop located on one face of the dimer, whereas two GDP molecules bind on the other face. Structure-guided mutagenesis shows that GDP binding is required for Ec FdhD function, demonstrating that the Ec FdhD–GDP complex structure is relevant for building a Mo- bis PGD binding model. Moreover, we show that the strictly conserved His171 residue located at one side of the tunnel is essential for Ec FdhD function. Our results support an overall mechanism by which the sulphurtransferase Ec FdhD ensures sulphuration of the Mo- bis PGD prior its insertion into FDH. In this model, sulphur is transported across the core of Ec FdhD from IscS to the molybdenum cofactor, thanks to the presence of a dynamic cysteine loop that reaches across the dimer. EcFdhD is a dimer that binds the molybdenum cofactor in vivo To characterize the function of Ec FdhD in molybdenum cofactor sulphuration, the ability of Ec FdhD to interact with Mo- bis PGD was investigated. First, Ec FdhD was purified by affinity chromatography as a dimer as deduced from gel filtration and dynamic light scattering analysis. The hydrodynamic radius of Ec FdhD in solution is 3.63±0.43 nm and its molecular mass is estimated at 68.7±8.2 kDa, which is compatible with a dimeric form of Ec FdhD ( Supplementary Fig. 1a ). The purified protein is coloured brownish pink and ultraviolet–visible absorption spectroscopy reveals the presence of absorption bands between 330 and 450 nm ( Supplementary Fig. 1b ). The absorption around 400 nm may be attributed to the ene-dithiolate-to-molybdenum charge transfer band [16] . 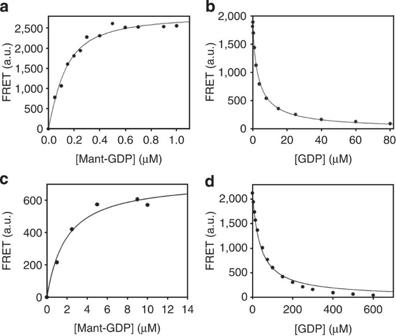Figure 1: GDP binding to EcFdhD. Binding properties ofEcFdhD (a,b) and of the double variantEcFdhDS240D/F260D(c,d). (a) FRET emission as a function of added Mant-GDP. The protein concentration is 0.1 μM. The line is a fit (see Methods) indicating a dissociation constantKM≈76 nM. (b) displacement of Mant-GDP (present at a concentration of 0.4 μM) as a function of added GDP. Protein concentration=0.4 μM. The line is a fit (see Methods) yieldingR≈0.11 for the ratio of dissociation constants. (c) same as (a); the fit yieldsKM≈1.9 μM. (d) same as (b), with Mant-GDP concentration=7.5 μM, yieldingR≈0.20. To further characterize the purified Ec FdhD protein, the molybdenum content and the stable oxidation product derived from the cofactor (the so-called formA-dephospho) were quantified by inductively coupled plasma mass spectrometry (ICP-MS) and high-performance liquid chromatography (HPLC) detection, respectively ( Supplementary Table 1 ). ICP-MS analysis revealed that 3.4% of the purified Ec FdhD contains molybdenum. The same protein fraction showed an average formA-dephospho saturation of about 5.6%, indicating that all cofactors bound to Ec FdhD contains molybdenum, since an Mo to formA-dephospho ratio of 1:2 is expected in Mo- bis PGD. Ec FdhD binds GDP with high affinity Because Mo- bis PGD is not available in its free form, its GDP moiety was chosen as a surrogate for studying its interaction with Ec FdhD using fluorescence spectroscopy. Figure 1a shows the binding of N -methylanthraniloyl (Mant)-GDP, a fluorescent analogue of GDP, monitored from the FRET signal of Mant sensitized by tryptophan. The dissociation constant is estimated from a fit using equation 4 (Methods). From this and other experiments at various concentrations of Ec FdhD, we obtained a mean value K M ≈76±25 nM. To obtain the dissociation constant of GDP, we monitored the displacement of Mant-GDP as a function of added GDP ( Fig. 1b ). A fit using equation 8 (Methods) yields the ratio of dissociation constants R ≈0.11 (meaning that the affinity for Mant-GDP is about 10-fold that for GDP). Combining the two pieces of information, we estimate the dissociation constant for GDP as K G ≈364 nM. We conclude that Ec FdhD possesses a high affinity for GDP. Figure 1: GDP binding to EcFdhD. Binding properties of Ec FdhD ( a , b ) and of the double variant Ec FdhD S240D/F260D ( c , d ). ( a ) FRET emission as a function of added Mant-GDP. The protein concentration is 0.1 μM. The line is a fit (see Methods) indicating a dissociation constant K M ≈76 nM. ( b ) displacement of Mant-GDP (present at a concentration of 0.4 μM) as a function of added GDP. Protein concentration=0.4 μM. The line is a fit (see Methods) yielding R ≈0.11 for the ratio of dissociation constants. ( c ) same as ( a ); the fit yields K M ≈1.9 μM. ( d ) same as ( b ), with Mant-GDP concentration=7.5 μM, yielding R ≈0.20. Full size image Structure of the Ec FdhD dimer and a disordered cysteine loop To gain insight into the structural basis underlying Mo- bis PGD binding by FdhD, the structure of Ec FdhD was solved in complex with GDP at a resolution of 2.8 Å ( Table 1 ). Each monomer of Ec FdhD folds into two domains, an N-terminal domain (NTD; residues 1–97) that is unique to the FdhD family, and a C-terminal domain (CTD; 147–277) bearing some structural homology with the cytidine deaminase fold ( Fig. 2a ). The NTD itself folds into two parts: the two first β strands build a single β-sheet that extends as a long arm (residue 15–40), with the remaining NTD folding as a four-stranded β-sheet wrapped around a single α-helix (α1). The cytidine deaminase fold of Ec FdhD consists of a six-stranded β-sheet that is packed on one side by a broken α-helix (α3-α3′) whereas the other side is packed with three α-helices (α4–α6). An α-helix (α2) followed by a long loop connects the NTD to the CTD in Ec FdhD (residue 98–146). This loop is partly disordered in each monomer with residues 113–131 not visible in the electron density map. Remarkably, this disordered part of the loop contains the pair of cysteine residues (Cys121–Cys124) shown to be functionally important [11] . The corresponding loop (residue 89–119) is also disordered in Dp FdhD, thereby suggesting a functional role for this disorder ( Supplementary Fig. 2 ). Interestingly, a careful analysis of the electron density map associated with Dp FdhD reveals that it is crystallized in such a way that there are two dimers in the asymmetric unit with four independent molecules instead of only one in the case of Ec FdhD, where the dimer is generated by a crystallographic twofold axis. This gives more freedom for each Dp FdhD monomer to adopt slightly different conformations. As a matter of fact, we found that the first dimer (AB) is symmetric and contains two disordered cysteine loops, whereas the second dimer (CD) is slightly asymmetric with 30 residues from the cysteine loop of monomer C entirely disordered, whereas the cysteine loop from monomer D is largely stabilized in the tunnel with only 6 residues still disordered ( Fig. 3 ). Table 1 Data collection and refinement statistics. 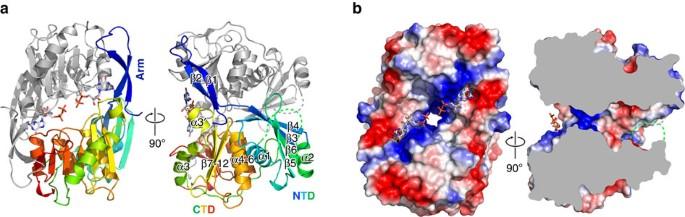Figure 2: Overall structure of theEcFdhD dimer in complex with GDP. (a) Secondary structure ofEcFdhD with one monomer coloured from blue (N-Terminus) to red (C-Terminus) and the other monomer coloured in grey. The GDP moiety is represented in stick. On the ‘front view’ (left) one can notice the arm that originates from one monomer and that packs against the adjacent monomer at the rim of the dimer. On the ‘side view’ (right) one can easily distinguish the N-Terminal domain (NTD: from β1 to α1), the C-Terminal domain (CTD: from α3 to β12) and the connector between the NTD and the CTD (α2 and the loop from α2 to α3). This connector is partly disordered and shown as a dotted line. This disordered part of the loop contains the residues Cys121 and Cys124. (b) Electrostatic surface representation ofEcFdhD in complex with GDP. The tunnel that crosses the center of the dimer is clearly visible. Full size table Figure 2: Overall structure of the Ec FdhD dimer in complex with GDP. ( a ) Secondary structure of Ec FdhD with one monomer coloured from blue (N-Terminus) to red (C-Terminus) and the other monomer coloured in grey. The GDP moiety is represented in stick. On the ‘front view’ (left) one can notice the arm that originates from one monomer and that packs against the adjacent monomer at the rim of the dimer. On the ‘side view’ (right) one can easily distinguish the N-Terminal domain (NTD: from β1 to α1), the C-Terminal domain (CTD: from α3 to β12) and the connector between the NTD and the CTD (α2 and the loop from α2 to α3). This connector is partly disordered and shown as a dotted line. This disordered part of the loop contains the residues Cys121 and Cys124. ( b ) Electrostatic surface representation of Ec FdhD in complex with GDP. The tunnel that crosses the center of the dimer is clearly visible. 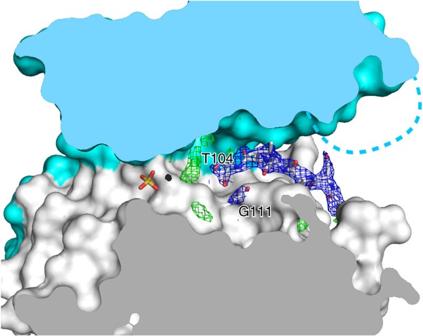Figure 3: The cysteine loops are differentially stabilized in the dimers of DpFdhD. Electron density map (blue: 2Fo-Fc contoured at 1σ and green: Fo-Fc contoured at 3σ) in the tunnel of oneDpFdhD dimer (pdb code 2pw9, unpublished). This electron density is clearly visible until Thr104 on one monomer and the only cysteine residue in the loop (Cys107) is still disordered. The solid surface corresponds to the residues that are resolved in both the AB and CD dimers. In this representation one monomer is coloured in grey and the other in light blue. Full size image Figure 3: The cysteine loops are differentially stabilized in the dimers of DpFdhD. Electron density map (blue: 2Fo-Fc contoured at 1σ and green: Fo-Fc contoured at 3σ) in the tunnel of one Dp FdhD dimer (pdb code 2pw9, unpublished). This electron density is clearly visible until Thr104 on one monomer and the only cysteine residue in the loop (Cys107) is still disordered. The solid surface corresponds to the residues that are resolved in both the AB and CD dimers. In this representation one monomer is coloured in grey and the other in light blue. Full size image As mentioned earlier, Ec FdhD is a dimer in solution ( Supplementary Fig. 1a ). This is confirmed by the crystal structure with a dimer generated by a crystallographic twofold axis. Dimerization of Ec FdhD buries 1,827 Å 2 on each monomer representing 15.6% of the total area on each subunit. This interface is also found in Dp FdhD with 1,900 Å 2 buried on each monomer (17.1% of the total surface area). Two parts of the protein mainly contribute to dimerization, a long arm formed by residues 21–41 in the NTD interact with residues 243–275 in the CTD of the adjacent monomer. This dimerization through two long arms located at the edge of the dimer creates a tunnel in its centre connecting two opposite faces of the dimer ( Fig. 2b ). At its most restricted part, the size of this tunnel is ~10 Å × 6 Å, which is sufficient for the putative transfer of reactive intermediates from one side to the other. Moreover, it is bordered by positively charged residues that are among the most highly conserved residues in the FdhD family (His171, Arg191, His192, Arg219 and Lys227; Supplementary Figs 2 and 3 ). The GDP binding site and its requirement for FDH activity The use of GDP during the crystallization process was intended to mimic the more complex substrate Mo- bis PGD. A clear electron density corresponding to two GDP molecules was observed at the interface of the dimer with residues involved in GDP binding coming from the arm in the NTD of one monomer and from the CTD of the adjacent monomer ( Fig. 4 and Supplementary Fig. 4 for a stereo view). The base moiety is the most stabilized part of the GDP molecule forming six putative hydrogen bonds with the protein (one such hydrogen bond involves the main chain of Leu166 and the other ones involve the side chains of Asp35, Arg25 and the side chain of Arg265 from the adjacent monomer). The nucleotide base is further stabilized by a stacking interaction with Phe260 from the other monomer. However, the ribose moiety of the GDP does not interact with the protein. Finally, a putative hydrogen bond with Ser240 and a salt bridge with Lys262 stabilize the first phosphate, whereas the second one is not involved in any interaction with the protein. 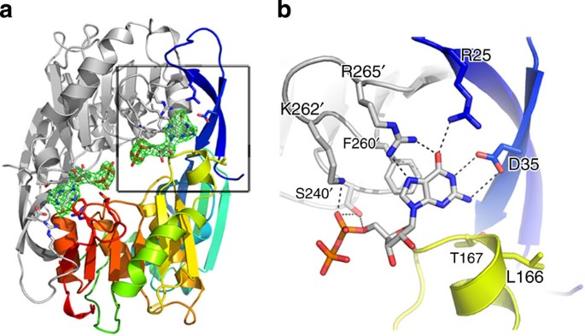Figure 4: GDP binding toEcFdhD. (a) Two molecules of GDP are bound on the same face of theEcFdhD dimer. The refined 2Fo-Fc electron density map is shown as a green mesh contoured at 1.5σ. (b) Details of the GDP binding site with all residues located 4 Å around the GDP shown in stick. These residues come from both monomers of the dimer. Figure 4: GDP binding to Ec FdhD. ( a ) Two molecules of GDP are bound on the same face of the Ec FdhD dimer. The refined 2Fo-Fc electron density map is shown as a green mesh contoured at 1.5σ. ( b ) Details of the GDP binding site with all residues located 4 Å around the GDP shown in stick. These residues come from both monomers of the dimer. Full size image To test the importance of nucleotide binding, a structure-guided mutagenesis of GDP coordinating residues was performed and the ability of variants to interact in vitro with GDP and to complement in vivo a fdhD deletion strain (Δ fdhD ) was assessed. On the basis of their high conservation ( Supplementary Fig. 2 ) and involvement in phosphate and base coordination, S240D and F260D variants were produced as single and double (S240D/F260D) variants. To obtain the dissociation constant of GDP, we proceeded as with Ec FdhD. For the Ec FdhD F260D , Ec FdhD S240D ( Supplementary Fig. 5a–d ) and Ec FdhD S240D/F260D ( Fig. 1c,d ) variants, the affinity for Mant-GDP was decreased with respect to the native protein, with K M ≈0.25, 2.06 and 1.9 μM, respectively. Combining with the chase experiments we estimate K G ≈5.6, 10.4 and 9.5 μM, respectively. Thus, the affinity to GDP is decreased about 30-fold in the variants, with no obvious enhancement in the double variant. One should notice that, if the binding of the Mo- bis PGD substrate is primarily controlled by the attachment of its two GDP groups, the 30-fold lower affinity to GDP is expected to correspond to a 900-fold decrease with regards to Mo- bis PGD. Indeed, the binding energy is the sum of the contribution from the two GDP binding sites, and the dissociation constant has an exponential dependence on the energy, K d =exp(−ΔG 0 /RT). If ΔG 0 (Mo- bis PGD)=2 × ΔG 0 (GDP), the dissociation constant for Mo- bis PGD varies as the square of the dissociation constant for binding an individual GDP. Thus, substitution of these conserved residues is found to drastically suppress the binding of the Mo- bis PGD. We proceeded to test the importance of these residues in vivo for FDH activity ( Fig. 5 ). All substitutions strongly impair the ability of Ec FdhD to complement the Δ fdhD strain with the Ec FdhD S240D/F260D variant being unable to give rise to FDH activity. In addition, two hybrid experiments showed that the Ec FdhD S240D/F260D variant retains the ability to interact with all its known partners FdhF, IscS and Ec FdhD ( Supplementary Fig. 6 ). This confirms that the role of these residues in the Ec FdhD ability to yield active FDH is linked to their involvement in GDP binding. 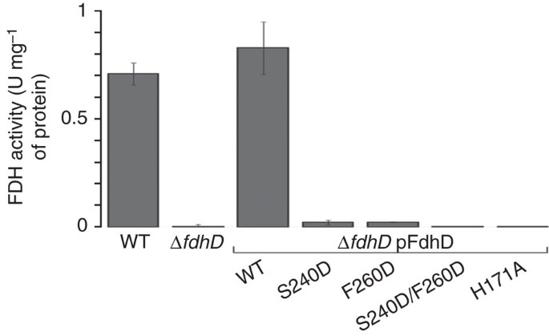Figure 5: Substitution of conserved residues ofEcFdhD severely impacts FDH activity. Wild-type (WT), ΔfdhDstrains transformed with an empty vector, or with pFdhD, pFdhDS240D, pFdhDF260D, pFdhDS240D/F260Dor pFdhDH171Awere grownin vivoin fermentative conditions. FDH activity was measured in crude extracts of each corresponding strains. One unit of FdhF activity is defined as the amount of μmol of formate reduced per minute per mg of total protein as described in materials and methods. FDH activity is expressed as means±s.d. and is a result from at least three independent experiments. Figure 5: Substitution of conserved residues of Ec FdhD severely impacts FDH activity. Wild-type (WT), Δ fdhD strains transformed with an empty vector, or with pFdhD, pFdhD S240D , pFdhD F260D , pFdhD S240D/F260D or pFdhD H171A were grown in vivo in fermentative conditions. FDH activity was measured in crude extracts of each corresponding strains. One unit of FdhF activity is defined as the amount of μmol of formate reduced per minute per mg of total protein as described in materials and methods. FDH activity is expressed as means±s.d. and is a result from at least three independent experiments. Full size image A model of Mo-bisPGD binding and functional validation A striking feature in the crystal structure of the Ec FdhD/GDP complex is the distance that separates the two GDP moieties in the dimeric complex. Indeed, this distance approximately corresponds to the distance observed in Mo- bis PGD-containing enzymes. For example, the distance between the two N 2 atoms of the guanine base is on average 32.9±1.2 Å in a selection of 13 independent Mo- bis PGD-containing enzymes, while it corresponds to 28.8 Å in Ec FdhD. Furthermore, the large solvent-exposed pocket that is present between the two GDP molecules in the Ec FdhD/GDP complex could accomodate such a large molecule. These two observations substantiate the copurification of Mo- bis PGD with Ec FdhD and prompted us to propose a model for Mo- bis PGD binding to Ec FdhD. Assuming that the two phosphate groups linking the guanosine and pyranopterin moieties could play the role of flexible linkers, the positions of the two GDP molecules were used as anchors and the two pyranopterin moieties were manually fitted in the solvent-exposed pocket. As a result, in our molecular model of Mo- bis PGD/ Ec FdhD, the hydrophobic face of the pyranopterin groups interacts with an apolar part of the solvent-exposed pocket on Ec FdhD ( Fig. 6 ). Notably, the 17 O atom (the oxo atom on the pterin moiety) of the Mo- bis PGD points towards the positively charged patches that are also facing the phosphate moieties. Modelling of Mo- bis PGD binding to Dp FdhD supports the same binding mode with the exception that the pocket is less solvent exposed and more charged ( Supplementary Fig. 7 ). These observations are in line with our current understanding of psychrophilic enzymes that favour electrostatic over hydrophobic interactions [17] . 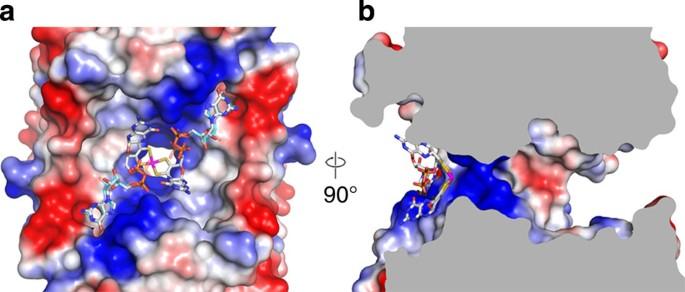Figure 6: A model of Mo-bisPGD binding onEcFdhD based on GDP positions. The electrostatic surface is shown together with the initial GDP molecules (in cyan-based coloured sticks and semitransparent rendering) and the Mo-bisPGD model (in white-based coloured sticks and solid rendering). Note that only the second phosphate is allowed to rotate so as to allow the pyranopterin moieties to interact deeper in the solvent exposed pocket ofEcFdhD. (a) Face view. (a) View after 90 °C rotation. Figure 6: A model of Mo- bis PGD binding on Ec FdhD based on GDP positions. The electrostatic surface is shown together with the initial GDP molecules (in cyan-based coloured sticks and semitransparent rendering) and the Mo- bis PGD model (in white-based coloured sticks and solid rendering). Note that only the second phosphate is allowed to rotate so as to allow the pyranopterin moieties to interact deeper in the solvent exposed pocket of Ec FdhD. ( a ) Face view. ( a ) View after 90 °C rotation. Full size image In our model, the molybdenum atom is surrounded by the most conserved residues of FdhD (His171, Arg191, His192, Ar219 and Lys227) ( Supplementary Figs 2 and 3 ), stressing that this region is crucial for the FdhD function. To test the importance of this region for the Ec FdhD function, one of these strictly conserved residues (His171) was substituted by an alanine residue. In fact, neither the ability of this variant to interact with its partners ( Supplementary Fig. 6 ) nor with GDP ( K G <60 nM) ( Supplementary Fig. 5e,f ) was affected by the substitution showing that the overall structural integrity was conserved. Most importantly, however, the Ec FdhD H171A variant is unable to promote FDH activity ( Fig. 5 ). The copurification of Ec FdhD with molybdenum cofactor to a similar extent as measured in R. capsulatus FdsC [15] confirms the ability of Ec FdhD to protect the unstable and air-sensitive cofactor, suggesting that FdhD plays the role of a chaperone. We further found that Ec FdhD can bind with high affinity to GDP alone, a building block used twice in the more complex Mo- bis PGD cofactor. The crystal structure of Ec FdhD in complex with GDP presented here—as well as the structure of Dp FdhD in its apo form (PDB 2PW9; unpublished)—possess four important features: (1) the protein exists as a dimer both in solution and in the crystals; (2) a small tunnel connects two, otherwise opposite, faces in all dimers; (3) one face of the dimer displays two disordered loops—called cysteine loops— that contain two functionally important cysteine residues (Cys121 and Cys124) and; (4) two molecules of GDP could be stabilized on the opposite face of the dimer in a conformation that allowed us to propose a model for the binding of the more complex Mo- bis PGD substrate. The fact that the cysteine loops can adopt different conformations and can be partially stabilized in the ‘tunnel’ suggests that they are dynamic and could easily shuttle a reactive intermediate derived from sulphur. Sequence alignment analysis reveals that in a few instances there is one or no cysteine residues in the cysteine loop ( Supplementary Fig. 2 ). A typical example is Dp FdhD that possesses a single cysteine residue equivalent to the E. coli Cys121. In some archaeal FdhD sequences there are no conserved cysteine residue. For example, in the euryarchaeota Methanococcus maripaludis , the protein has conserved the ability to bind the Mo- bis PGD as judged by the conservation of the residues involved in GDP binding, but has likely lost the ability to sulphurate it as judged by the absence of the catalytic cysteine loop. It is noteworthy that this archaeon appears to lack a cysteine desulphurases [18] , which raise the possibility that the FdhD homologue functions as a chaperone only and does not participate in the sulphuration of Mo- bis PGD. In the case of the R. capsulatus FdsC, the sequence harbours two cysteine residues within the loop, but their substitutions for alanine residues did not impair R. capsulatus FDH activity in E. coli [15] . FdsC was shown to bind Mo- bis PGD, consistent with conservation of the residues involved in Mo- bis PGD binding identified in our study. We propose that FdsC mainly functions as a chaperone in the Rc FDH maturation and, in contrast to Ec FdhD, is not involved in cofactor sulphuration. This could either be because another protein fulfills this role in E. coli , or simply because the cofactor does not require sulphuration—a situation that might well exist, since it is not known whether all FDH proteins depend on a sulphurated Mo- bis PGD. As previously reported [19] , the cysteine desulphurase IscS proceeds to a reductive elimination of sulphur from L -cysteine in the form of a cysteine–persulphide intermediate. So far, the precise reaction mechanism by which the inorganic sulphur of the cysteine–persulphide intermediate is transferred to the molybdenum atom of a bound cofactor remains unknown. Such a situation does not only applies to FdhD, but also to members of the xanthine oxidase family from both eukaryotes and prokaryotes, where a dedicated protein is in charge of molybdenum cofactor sulphuration prior to its insertion into the target enzymes [16] , [20] , [21] . It was also reported that sulphur transfer by persulphide chemistry may occur through two chemically reasonable routes [22] , [23] . In the first, the terminal sulphur of the persulphide group bound on the catalytic cysteine residue is released by a second active site cysteine. The resulting ‘free’ bisulphide is presumably sequestered and serves as the immediate thiolating agent of the substrate. In the second route, the persulphide group carries a nucleophilic attack the activated substrate and generates a disulphide bond that links the enzyme to its substrate. A second active site cysteine residue then allows release of the sulphurated substrate. Our data can accommodate either of these routes, as the presence of a molecular tunnel in FdhD very likely protects the reactive persulphide group intermediate from the bulk solution. In both routes, the most conserved residues of FdhD (His171, Arg191, His192, Ar219 and Lys227 in Ec FdhD) would assist sulphur transfer as they are located at one side of the tunnel and His171 mutagenesis abolishes FDH activity ( Fig. 5 ). In conclusion, our results provide a plausible structural basis for the sulphurtransferase activity of Ec FdhD, suggesting a sophisticated mechanism by which the sulphur is transported from IscS on one side of the FdhD dimer to the molybdenum cofactor on the other side prior to its final insertion into FDH ( Supplementary Fig. 8 ). The mechanism we propose can serve as a basis for a better understanding of the molecular details underlying sulphuration of the molybdenum cofactor at play in members of the xanthine oxidase family. Bacterial strains and growth conditions The E. coli strains used in this work are described in Supplementary Table 2 . BTH101 was used as recipient strain for two-hybrid assays. Shuffle T7 strain (New England biolabs) was employed for overexpression of fdhD and its variants using pET22b-type expression plasmids (Novagen). Growth conditions for overproduction of Ec FdhD and its variants were as in ref. 11 . For ICP-MS and FormA-dephospho quantification of Mo- bis PGD, shuffle T7 strain transformed with pET22-FdhD was grown in medium supplemented with Na 2 MoO 4 (1 mM). When required, the appropriate antibiotics were added. Cloning and mutagenesis The plasmids used in this work are described in Supplementary Table 2 . Site-specific mutagenesis was performed as in ref. 24 with primers 622: 5′- GTGCGGCGTAGAGATTTTGTTTGCGGTGGATGC -3′ and 623: 5′- CACTTCTACAGCAAGCGTGGTCGCGGCATCCAC -3′ to substitute codon encoding serine 240 of Ec FdhD into aspartate codon, with primers 626: 5′- GAGCGCTGTAATCTGACACTGGTAGGTGATTG -3′ and 627: 5′- CGTTGCCCGACCCGGTTTACAATCACC -3′ to substitute codon encoding phenylanine 260 of Ec FdhD into aspartate codon and with primers 575: 5′- CAGCCAGTGGGGCAACTGACTGGTTGTACTGCAGC -3′ and 576: 5′- CCAGTTCGCCAGATGGCAACATCCAGGCAGCGGCTGCA -3′ to substitute codon encoding histidine 171 of Ec FdhD into alanine codon. Dynamic light scattering The purified Ec FdhD protein was analysed by DLS assays carried out through a laser wavelength of 633 nm, using a Zetasizer nano S (Malvern instruments) molecular-sizing instrument equipped with a Peltier system for temperature control. Solutions of proteins were centrifuged at 15,000 g for 20 min at 4 °C, and the supernatant filtered through a 0.22 μm filter (Millipore) and added to the cuvette. The hydrodynamic parameters were measured at 20 mM Tris-HCl, pH 7.4, 200 mM NaCl, at a protein concentration of 3 μM of Ec FdhD. Hydrodynamic radius and molecular weight were determined from the intensity correlation function using the Dynamics V.6 software. The experiments were performed with an average of 15 acquisitions. Chemical detection of Mo- bis PGD For analysis of Mo- bis PGD and eventually bound Mo-MPT, either 500 or 1,000 pmol of Ec FdhD in 0.4 ml 0.1 M Tris/HCl, pH 7.2 were subjected to acidic oxidation by addition of 50 μl oxidation solution (stock: 914 μl 1% I 2 /KI and 86 μl 37% HCl) and incubation in the dark for 30 min at 95 °C to convert MPT moieties of cofactors into FormA. After centrifugation for 5 min at 21,000 g , the supernatant was transferred to new 1.5-ml tubes and mixed with 56 μl 1% ascorbic acid. Subsequently, 200 μl 1 M unbuffered Tris, 13 μl 1 M MgCl 2 and 0.5 μl alkaline phosphatase (Roche) were added and incubated overnight at room temperature to remove the terminal phosphate group of MPT-derived FormA, thereby yielding FormA-dephospho. Samples were again centrifuged for 5 min at 21,000 g and subjected to anion exchange chromatography on Q-sepharose matrix (GE Healthcare) equilibrated with 1 M ammonium acetate. After washing with water, samples were loaded onto columns and MPT-based FormA-dephospho was eluted in 800 μl 10 mM acetic acid after washing columns with water. To purify oxidized Mo- bis PGD as FormA-dephospho, the same columns were washed with 3 ml 10 mM acetic acid to remove eventually persisting MPT/FormA-dephospho and elution was performed in 800 μl 50 mM HCl. Subsequently, the elution fraction was split into two aliquots of 400 μl and each aliquot was supplemented with 25.2 μl 1 M unbuffered Tris, 5.25 μl 1 M MgCl 2 and 1 μl phosphodiesterase I from rattle snake (1 U μl −1 ; Biomol, Hamburg, Germany) to separate the pterin and nucleotide moieties in oxidized Mo- bis PGD. Reactions were incubated overnight at room temperature in the dark. After inactivation of phosphodiesterase I by heat treatment (96 °C for 5 min), samples were cooled on ice for 3 min and dephosphorylated by addition of 10.5 μl 1 M unbuffered Tris and 2 μl alkaline phosphatase and again incubated overnight at room temperature in the dark. After all, the two aliquots were combined and subjected to anion exchange chromatography on Q-sepharose matrix, and elution of FormA-dephospho derived from Mo- bis PGD was performed as described for MPT. Finally, HPLC analysis was performed as described in ref. 14 . Metal analysis Metal analysis of purified Ec FdhD was performed using ICP-MS. Protein samples were wet-ashed in a 1:5 mixture with 65% v/v nitric acid, for 2 days. Samples were then diluted with 3 ml of ultrapure water 18 MΩ. The solutions obtained were then analysed in triplicate by ICP-MS using a Thermo Series II ICP/MS apparatus (Thermo-Electron, Les Ulis, France). As reference, a multielement standard solution (SCP Sciences, Canada) was used. Metal concentrations were finally determined using Plasmalab software (Thermo-Electron, Les Ulis, France). Bioinformatics A multiple alignment sequences was done with Jalview [25] and with the following FdhD like sequences from E. coli (NCBI Reference Sequence: NP_418331.1), from R. capsulatus (YP_003579165.1), from D. psychrophila (YP_065513.1) from Cupriavidus taiwanensis (YP_002006409.1), from Wolinella succinogenes (NP_906299.1), from Desulfitobacterium hafniense (YP_520523.1), from Streptomyces coelicolor (NP_630639.1), from Mucilaginibacter paludis (WP_008504089.1), from Lyngbya sp (WP_009784382.1), from Nostoc punctiforme (YP_001864330.1), from M. maripaludis (YP_001549485.1) and from Thermofilum pendens (YP_920659.1). Bacterial two-hybrid assay Protein interactions were detected using a bacterial two-hybrid approach as described previously [11] , [26] . Briefly, protein interactions were estimated by measurement of β-galactosidase activity in cells grown to mid-log phase in anaerobiosis at 30 °C in L-broth medium supplemented with 0.5 mM isopropyl-1-thio-β- D -galactopyranoside (IPTG), HCOONa (12.5 mM), Na 2 MoO 4 (2 μM) and Na 2 SeO 3 (2 μM). Statistical analysis All data are expressed as means±s.d. Data for each experiment were acquired from at least three independent experiments. Protein purification Ec FdhD purification and its variants were performed by nickel-affinity chromatography as described in ref. 11 . For the gel filtration, the Superdex 200 column (1 × 30 cm) was equilibrated with buffer containing Tris-HCl 20 mM pH 7.2, NaCl 150 mM. 50 μl of purified Ec FdhD at 240 μM was applied to the column. The enzyme was then eluted in 0.5-ml fractions with 1 column volume of the same buffer. FDH activity Crude extracts of strains grown anaerobically in L-broth medium supplemented with glucose (1%), HCOONa (12.5 mM), Na 2 MoO 4 (2 μM) and Na 2 O 3 Se (2 μM) were used to measure FDH activity of Ec FdhF by following the reduction of benzyl viologen (BV) spectrophotometrically at 600 nm coupled to the oxidation of sodium formate at 37 °C in an anaerobic glove box (100% N 2 ) [27] . FDH activity is expressed in μmol of formate reduced min −1 per mg of protein. Fluorescence measurements All experiments were performed at room temperature using a SAFAS flx-Xenius 5,117 spectrofluorimeter. All spectra were corrected for buffer fluorescence. Fluorescence measurements were routinely carried out after dilution of Ec FdhD or its variants and equilibration for 2 min in 2 ml of a buffer containing 25 mM HEPES-KOH (pH 7). The binding of GDP to Ec FdhD or its variants could not be monitored directly and was estimated using the fluorescent analogue Mant-GDP (Molecular probes). When the protein binds Mant-GDP, an efficient excitation transfer is observed from tryptophan to Mant. The FRET signal obtained in this manner (excitation at 282 nm, emission integrated in the 384–490 nm region) corresponds to the amount of the complex of the Ec FdhD or its variants with Mant-GDP (denoted [FM] in the treatment given below). In a separate series of experiments, the displacement of a saturating concentration of Mant-GDP by added GDP was studied, which, as shown below, yields the ratio of dissociation constants of both ligands. Theoretical functions for binding and displacement of Mant-GDP We denote as [ F ], [ G ], [ M ] the concentrations of the free forms of Ec FdhD or its variants, of GDP and of Mant-GDP, respectively. The complexed forms are noted [ FG ] and [ FM ], and the total amount of each species (free form+complex) is indicated with subscript t . In the presence of the sole ligand M , one has the relations: where K M is the dissociation constant for Mant-GDP. Combining these equations one obtains a trinomial, with the root: The above function was used for fitting the experimental data for [ FM ] as a function of [ M ] t (added Mant-GDP) with K M as an adjustable parameter. A meaningful estimate of K M cannot be obtained when [ F ] t >> K M . In the experiments with Ec FdhD, Ec FdhD S240D , Ec FdhD F260D , Ec FdhD H171A , Ec FdhD C121A/C124A used at concentrations [ F ] t above 0.2 μM, there was clear indication that a significant fraction of protein was inactive, since the saturation occurred at Mant-GDP concentrations <[ F ] t . This did not occur at lower protein concentrations, as shown by fitting with equation 4 with [ F ] t as a free parameter (in addition to K M ). Thus, experiments of Fig. 1a,c and Supplementary Fig. 5a,c,e,g were run at [ F ] t =0.1 μM. For the displacement experiments, we used a nearly saturating concentration of Mant-GDP so that, irrespective of the amount of GDP, the amount of free enzyme [F] is negligible. Then, The dissociation equilibrium for GDP ( K G ) writes: Combining the above equations, one obtains a second order equation: where a = R −1, b =[ M ] t +[ F ] t + R ([ G ] t −[ F ] t ) and c =−[ F ] t [ M ] t . R≡ K M / K G is the ratio of dissociation constants. The relevant root is: Equation 8 was used to fit the experiments monitoring the amount of [FM] from the FRET signal, as a function of the added GDP ([ G t ]), in the presence of a fixed concentration of Mant-GDP ([ M t ]). Structure determination For crystallization, Ec FdhD was desalted in the last purification buffer [11] except the glycerol was omitted. GDP was then added to a final concentration of 10 mM and the complex was concentrated to 5 mg ml −1 . Crystals were obtained in a sitting drop setup by mixing 0.5 μl of protein with an equal volume of a mother liquor made of 2.2 M ammonium sulphate and 0.2 M sodium nitrate. Crystals appeared within a day and reached their final size within a few days. For cryoprotection crystals were gradually transferred in a mother liquor supplemented with 30% glycerol. Data were collected at beamline ID29 (ESRF) and processed using Mosflm and Scala from the CCP4 suite [28] . The structure of E. coli FdhD was solved by molecular replacement using the structure given in the PDB entry 2PW9 as a searched model and the programme Balbes [29] . PDB entry 2PW9 depict the 3D structure of a formate dehydrogenase accessory protein from D. psychrophila (30% identity with E. coli FdhD over 246 residues). One molecule per asymmetric unit was found and the dimer of Ec FdhD is generated through a crystallographic symmetry axis. The structure was then refined with the programme phenix.refine with manual building using the programme COOT [30] . From the first refinement cycles, additional electron density corresponding to the GDP became visible. The quality of the model was validated using the programs Procheck and SFcheck. Figures were made using the Pymol programme and surface area calculations were calculated with the PISA server. How to cite this article : Arnoux, P. et al . Sulphur shuttling across a chaperone during molybdenum cofactor maturation. Nat. Commun. 6:6148 doi: 10.1038/ncomms7148 (2015). Accession codes: The atomic coordinates and structure factors have been deposited in the Protein Data Bank under accession code 4PDE .